Optical focusing deep inside dynamic scattering media with near-infrared time-reversed ultrasonically encoded (TRUE) light Focusing light deep inside living tissue has not been achieved despite its promise to play a central role in biomedical imaging, optical manipulation and therapy. To address this challenge, internal-guide-star-based wavefront engineering techniques—for example, time-reversed ultrasonically encoded (TRUE) optical focusing—were developed. The speeds of these techniques, however, were limited to no greater than 1 Hz, preventing them from in vivo applications. Here we improve the speed of optical focusing deep inside scattering media by two orders of magnitude, and focus diffuse light inside a dynamic scattering medium having a speckle correlation time as short as 5.6 ms, typical of living tissue. By imaging a target, we demonstrate the first focusing of diffuse light inside a dynamic scattering medium containing living tissue. Since the achieved focusing speed approaches the tissue decorrelation rate, this work is an important step towards in vivo deep tissue noninvasive optical imaging, optogenetics and photodynamic therapy. In biomedicine, light focusing plays a critical role in imaging molecules with high resolution and sensitivity [1] , [2] , [3] , and in delivering optical energy precisely at a targeted position to perform optical manipulation [4] , stimulation [5] and microsurgery [6] . However, in biological tissue, photons are scattered by wavelength-scale refractive index inhomogeneities. As a result, it becomes infeasible to focus light with lenses beyond approximately one transport mean free path [7] , [8] , [9] , [10] ( l t ’, corresponding to ~1 mm in human skin), which fundamentally limits the imaging depth of conventional optical microscopy, such as confocal microscopy, two-photon microscopy and optical coherence tomography. To achieve the highly desired goal of focusing randomly scattered light deep inside scattering media, two categories of techniques have recently been developed: internal-guide-star-based wavefront shaping [11] , [12] , [13] , [14] , [15] , [16] , [17] and time-reversed ultrasonically encoded (TRUE) optical focusing [10] , [18] , [19] , [20] , [21] , [22] , [23] , [24] , [25] , [26] . In wavefront shaping [27] , the phase of the light incident on a scattering medium is shaped by an addressable spatial light modulator (SLM) to compensate for the scattering-induced phase distortions. To focus light inside scattering media, an internal guide star is needed at the targeted location. By optimizing the feedback signal from the guide star iteratively, an optimum phase pattern is determined that enables scattered light propagating along different paths to interfere constructively at the targeted location, thus forming a focus. So far, embedded fluorescent particles [11] and acoustic waves [12] , [13] , [14] , [15] , [16] , [17] have been employed as the internal guide stars. Although great effort has been made to speed up the wavefront-shaping process [28] , [29] , obtaining the optimum phase pattern is usually time-consuming, due to its iterative nature. The required number of independent control elements increases quadratically with depth (see Supplementary Note 1 ), making the method even slower for deep-tissue applications. TRUE optical focusing, an alternative technology to focus light deep inside scattering media, is inherently faster. It combines focused ultrasonic modulation [30] , [31] , [32] , [33] with optical phase conjugation [34] (OPC). In this technique, a phase conjugate mirror (PCM) records and then time-reverses the ultrasound-modulated light emitted from an ultrasonic focus, thereby achieving optical focusing (see Fig. 1a ). PCM has been implemented using either analogue photorefractive materials [10] , [18] , [19] , [20] , [21] , [22] , [23] , or a digital addressable SLM in precise alignment with a camera [24] , [25] , [26] . Unlike wavefront shaping, TRUE focusing measures the desired phase map globally without iteration. Nonetheless, the speed of TRUE focusing has been limited to no greater than 1 Hz [19] , [24] , [25] , due either to the slow response of the photorefractive PCM for analogue TRUE [10] , [19] , [21] , or to the low speed of data acquisition, processing and transfer among the digital camera, the computer and the SLM for digital TRUE [24] , [25] . 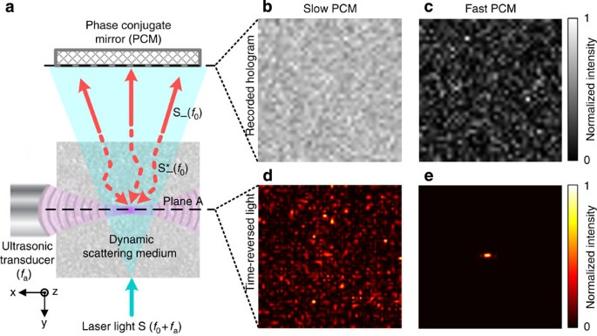Figure 1: The influence of phase conjugation speed on the quality of TRUE optical focusing. (a) Illustration of the TRUE focusing concept. Laser light S with a frequency off0+failluminates a scattering medium and a portion of the diffuse light traversing the acoustic focus is frequency-downshifted tof0(the frequency of the acoustic wave isfa). A PCM records the wavefront of these ultrasonically modulated light S−(f0) in a hologram and then phase-conjugates the light back to the ultrasonic focus, thereby forming a focus. Dashed arrows indicate time-reversed light. Plane A denotes thex–zplane intersecting the acoustic axis. (b,c) Simulated recorded holograms in a slow (b) and fast (c) PCM. Hologram blurring is clearly visible inbas a reduction in speckle contrast. (d,e) Simulated light intensity distribution on plane A by reading the hologram recorded in the slow (d) and fast (e) PCM. No focusing can be observed ind. All the images inb–ewere normalized by their own maximum values. S, sample light; S−, frequency-downshifted sample light (signal light);, time-reversed signal light; TRUE, time-reversed ultrasonically encoded. Figure 1: The influence of phase conjugation speed on the quality of TRUE optical focusing. ( a ) Illustration of the TRUE focusing concept. Laser light S with a frequency of f 0 + f a illuminates a scattering medium and a portion of the diffuse light traversing the acoustic focus is frequency-downshifted to f 0 (the frequency of the acoustic wave is f a ). A PCM records the wavefront of these ultrasonically modulated light S − ( f 0 ) in a hologram and then phase-conjugates the light back to the ultrasonic focus, thereby forming a focus. Dashed arrows indicate time-reversed light. Plane A denotes the x–z plane intersecting the acoustic axis. ( b , c ) Simulated recorded holograms in a slow ( b ) and fast ( c ) PCM. Hologram blurring is clearly visible in b as a reduction in speckle contrast. ( d , e ) Simulated light intensity distribution on plane A by reading the hologram recorded in the slow ( d ) and fast ( e ) PCM. No focusing can be observed in d . All the images in b – e were normalized by their own maximum values. S, sample light; S − , frequency-downshifted sample light (signal light); , time-reversed signal light; TRUE, time-reversed ultrasonically encoded. Full size image To date, these technologies have been confined to experimentation with static scattering media, such as ground glass diffusers, translucent tapes, tissue-mimicking phantoms and ex vivo biological tissue, whose speckle correlation times are greater than [24] 180 s. None have been applied to focusing light inside dynamic scattering media or living biological tissue. This restriction is because of the requirement that the deterministic property of light propagation in the scattering medium must be maintained during the course of focusing. In living biological tissue, displacement of scatterers due to breathing, blood flow and Brownian motion causes the speckle pattern [35] (a random interference pattern formed by coherent light after propagating through a scattering medium) to decorrelate, reducing the speckle correlation time to the order of 1 ms [36] , [37] , which further depends on the depth of interrogation. Thus, in TRUE optical focusing, if the PCM does not respond fast enough, a blurred hologram will be recorded ( Fig. 1b ). When this blurred hologram is read, no optical focus can be formed at the ultrasonic focal position ( Fig. 1d ). Therefore, in order to achieve optical focusing inside dynamic scattering media, the PCM (and the TRUE focusing system) must respond sufficiently fast, so that hologram recording and reading can be completed within the speckle correlation time ( Fig. 1c,e ). A similar requirement applies to wavefront-shaping-based focusing approaches, where the iterative measurements must be completed within the speckle correlation time. In this work, we present a solution to overcome the optical focusing challenges in nonstatic scattering media, by developing a high-speed TRUE focusing system with a 1% tellurium-doped tin thiohypodiphosphate (Sn 2 P 2 S 6 :Te 1%) photorefractive crystal (PRC) [38] , [39] , [40] as the PCM. The crystal is sensitive to light ~790-nm wavelength, making it particularly suitable for focusing light deep inside biological tissue, since the attenuation of near-infrared light in tissue is weaker than that of visible light [41] . More importantly, the crystal responds on the order of milliseconds under moderate optical illumination [38] , [39] , [40] (for example, 7 ms at 1 W cm −2 and 1.3 ms at 10 W cm −2 ), which is potentially fast enough to overcome the rapid speckle decorrelation caused by living tissue. Through direct visualization of the time-reversed light pattern, and by imaging an absorptive target embedded inside a dynamic scattering medium, we evaluate the TRUE focusing performance of our system at various speckle decorrelation rates. We confirm that our system is able to focus light inside a dynamic scattering medium having a speckle correlation time as short as 5.6 ms. The improved speed enables us to achieve the first optical focusing of diffuse light inside a scattering medium containing living biological tissue. Tissue-mimicking phantom experiments Here we demonstrated TRUE optical focusing inside a dynamic scattering medium composed of an intralipid-gelatin phantom (IP, thickness=1.5 mm, reduced scattering coefficient=0.98 mm −1 ) and a ground glass diffuser (see Methods for details on sample preparation). An absorptive target was sandwiched between the two scattering media to mimic an optical heterogeneity, such as a tumour, inside tissue. By translating the IP at different speeds, speckle patterns with different speckle correlation times ( τ c ) were created. The set-up illustrated in Fig. 2a was used to characterize the dependence of the speckle correlation time on the phantom movement speed. As shown, the diffuse light passing through the diffuser and the IP was collected by a lens L, and concentrated on the PRC. To measure the speckle patterns on the front surface of the PRC, light was reflected by a mirror and directed to a finite-conjugate objective whose object plane was a mirrored plane of the surface of the PRC. When the IP was moved at different speeds along the x axis, the corresponding speckle patterns were magnified by the objective and recorded on a CMOS camera (see Methods). Then, we calculated the correlation coefficients between the first and each of the ensuing frames of the recorded patterns. By fitting the speckle correlation coefficient versus time using a Gaussian function [35] , [42] , we obtained τ c , defined as the time during which the correlation coefficient decreased to 1/ e 2 or 13.5%, at a given phantom movement speed. As an example, Fig. 2b shows the speckle correlation coefficient as a function of time when the phantom was moved at v =0.010 mm s −1 , from which τ c =60 ms was determined. The relationship between the speckle correlation time and the phantom movement speed is shown in Fig. 2c . Theoretically, τ c = d b / v , where d b is the expected size of the speckle grains back-projected from the camera to the surface of the IP through lens L and the objective. From its definition, d b = d /( M 1 M 2 ), where M 1 (=2.8, simulated by Zemax, Zemax, LLC, USA) and M 2 (=40) are the magnifications of L and the objective, respectively, and d is the expected speckle size on the camera ( d = λl / D where λ is the optical wavelength, l (150 mm) is the distance between L and the PRC, and D (75 mm) is the aperture size of L). From the fitted curve in Fig. 2c , d b =0.56±0.01 μm ( R 2 =0.999), which is close to its theoretical value of λl /( DM 1 M 2 )=0.57 μm. The value of τ c at different speeds can therefore be estimated from τ c =0.56 v −1 [ms] (the unit of v is mm s −1 ), especially when v >0.040 mm s −1 (for those speeds, it was impossible to measure τ c accurately with the current set-up, since the frame rate of the camera was limited to 208 frames per second (fps)). 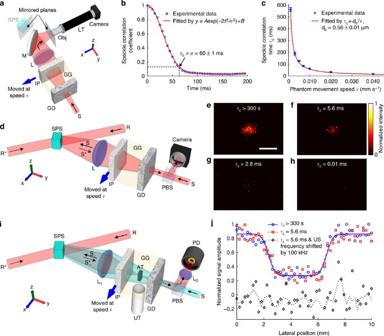Figure 2: TRUE optical focusing inside a dynamic scattering medium containing a tissue-mimicking phantom. (a) Schematic of the set-up for characterizing the relationship between the speckle correlation time (τc) and the phantom movement speed. The front surface of the crystal and the object plane of the objective were mirrored planes. (b) The speckle correlation coefficient as a function of time when the phantom was moved at 0.010 mm s−1.τc=60 ms was determined for this speed. (c) The relationship between the speckle correlation time and the phantom movement speed. Error bar shows the s.e. ofτcmeasured when light illuminated three different locations on the intralipid–gelatin phantom. (d) Schematic of the set-up for evaluating the quality of the time-reversed light at various sample decorrelation rates. (e–g) The time-reversed light pattern when the intralipid–gelatin phantom was static (τc>300 s,e), moved at 0.100 mm s−1(τc=5.6 ms,f) and at 0.200 mm s−1(τc=2.8 ms,g). (h) No time-reversed light was observed when the frequency of S was shifted by 100 kHz (τc=0.01 ms). All the images ine–hwere normalized by their own maximum values. (i) Schematic of the set-up for imaging an absorptive target with TRUE light. The target was scanned along thexdirection. (j) One-dimensional images of the target acquired under different conditions. The circles, squares and diamonds denote experimental data. The solid and dashed lines denote curve fitting of the experimental data. The dotted line denotes the four-point moving average of the experimental data. AT, absorptive target; GD, ground glass diffuser; GG, gelatin gel; IP, intralipid–gelatin phantom; L, lens; LT, lens tube; M, mirror; Obj, Objective; PBS, polarizing beamsplitter; PD, photodiode; R, reference beam; R*, reading beam, phase conjugate to R; S, sample light; S−, frequency-downshifted sample light (signal light);, time-reversed signal light; SPS, Sn2P2S6:Te 1% photorefractive crystal; TRUE, time-reversed ultrasonically encoded; US, ultrasound; UT, ultrasonic transducer. Scale bar, 1 mm. Figure 2: TRUE optical focusing inside a dynamic scattering medium containing a tissue-mimicking phantom. ( a ) Schematic of the set-up for characterizing the relationship between the speckle correlation time ( τ c ) and the phantom movement speed. The front surface of the crystal and the object plane of the objective were mirrored planes. ( b ) The speckle correlation coefficient as a function of time when the phantom was moved at 0.010 mm s −1 . τ c =60 ms was determined for this speed. ( c ) The relationship between the speckle correlation time and the phantom movement speed. Error bar shows the s.e. of τ c measured when light illuminated three different locations on the intralipid–gelatin phantom. ( d ) Schematic of the set-up for evaluating the quality of the time-reversed light at various sample decorrelation rates. ( e – g ) The time-reversed light pattern when the intralipid–gelatin phantom was static ( τ c >300 s, e ), moved at 0.100 mm s −1 ( τ c =5.6 ms, f ) and at 0.200 mm s −1 ( τ c =2.8 ms, g ). ( h ) No time-reversed light was observed when the frequency of S was shifted by 100 kHz ( τ c =0.01 ms). All the images in e – h were normalized by their own maximum values. ( i ) Schematic of the set-up for imaging an absorptive target with TRUE light. The target was scanned along the x direction. ( j ) One-dimensional images of the target acquired under different conditions. The circles, squares and diamonds denote experimental data. The solid and dashed lines denote curve fitting of the experimental data. The dotted line denotes the four-point moving average of the experimental data. AT, absorptive target; GD, ground glass diffuser; GG, gelatin gel; IP, intralipid–gelatin phantom; L, lens; LT, lens tube; M, mirror; Obj, Objective; PBS, polarizing beamsplitter; PD, photodiode; R, reference beam; R*, reading beam, phase conjugate to R; S, sample light; S − , frequency-downshifted sample light (signal light); , time-reversed signal light; SPS, Sn 2 P 2 S 6 :Te 1% photorefractive crystal; TRUE, time-reversed ultrasonically encoded; US, ultrasound; UT, ultrasonic transducer. Scale bar, 1 mm. Full size image To evaluate the limiting speed of our system in achieving OPC, we used the set-up illustrated in Fig. 2d to directly visualize the time-reversed light patterns at various sample decorrelation rates. The diffuse sample light S passing through the scattering medium interfered with a reference beam R (plane wave, with the same optical frequency as that of S) for 10 ms and wrote a volumetric hologram inside the PRC. Then, S and R were blocked, and a reading beam R*, conjugate to R, was applied to illuminate the PRC for 2 ms, generating a phase-conjugated copy of S, that is, the time-reversed light S*, which was monitored by a CMOS camera in real time. The intensity distributions of S* when the IP was static ( τ c >300 s), moved at v =0.100 mm s −1 ( τ c =5.6 ms) and at v =0.200 mm s −1 ( τ c =2.8 ms) are shown in Fig. 2e–g . To quantify the phase conjugation quality, we calculated the ratio R I between the averaged light intensities within ( ) and outside ( ) the targeted region of the phase-conjugated light (the region was determined when τ c >300 s, as shown in Fig. 2e ). To determine the limiting speed of our system in achieving OPC, we identified the shortest speckle correlation time at which was satisfied (where σ ( I out ) is the s.d. of the background light intensity outside the targeted region). Phase conjugation could be achieved when τ c =5.6 ms ( Fig. 2f ), although at a degraded quality ( R I =114) compared with that when τ c >300 s ( Fig. 2e , R I =287). In contrast, when τ c =2.8 ms ( Fig. 2g ), R I dropped to 5. Compared with the phase-conjugated light pattern when τ c =5.6 ms, the diffracted light was much less localized when τ c =2.8 ms, and it was coupled into a stronger background, suggesting that the PRC could not produce time-reversed light with good fidelity. When the frequency of S was detuned by 100 kHz (by using acousto-optic modulators (AOMs), corresponding to τ c =0.01 ms), no time-reversed light was observed ( Fig. 2h , R I =0.7). This result was expected, since the interference pattern decorrelated at a speed (100 kHz) greater than the response speed of the PRC and the hologram was washed out. The shortest speckle correlation time our system could tolerate defined with was between 2.8 and 5.6 ms. We further demonstrated that TRUE focusing and imaging could be accomplished when τ c =5.6 ms using the set-up illustrated in Fig. 2i . In this experiment, light S with a frequency of f 0 + f a ( f 0 was the laser frequency and f a (3.5 MHz) was a frequency detuning applied by AOMs) illuminated the scattering media (see Methods and Supplementary Fig. 1 for a complete schematic of the experimental set-up). The frequency of a portion of the diffuse light traversing the ultrasonic focus was downshifted to f 0 because of the acousto-optic effect [31] , [32] (the frequency of the ultrasonic wave was f a =3.5 MHz). These photons (the frequency-downshifted sample light S − , also called signal light) contributed to a stable hologram in the PRC by interfering with R, whose frequency was also f 0 . Thereby, the recorded hologram corresponded to a wavefront emanating from the ultrasonic focus. When the hologram was then read by R* (with a frequency of f 0 ), the time-reversed signal light was generated and converged back to the acoustic focus. A photodiode was used to sample that came out of the diffuser, and the photodiode outputs corresponding to light diffracted from the holograms that were recorded when the focused ultrasonic modulation was on and off are shown in Supplementary Fig. 2 , when the IP was moved at v =0.100 mm s −1 ( τ c =5.6 ms). The positive difference between the maximum signal amplitudes at the on and off states confirmed effective TRUE focusing when τ c =5.6 ms. Such a positive difference could no longer be observed repetitively when the frequency of the focused ultrasonic modulation was downshifted by 100 kHz to f a ′=3.4 MHz (see Supplementary Fig. 2b ). This result was expected, since the interference pattern of the ultrasonically encoded light and the reference beam decorrelated too fast (at f S− − f R =[( f 0 + f a )− f a ′]− f 0 = f a − f a ′=3.5−3.4 MHz=0.1 MHz, and f S+ − f R =[( f 0 + f a )+ f a ′]− f 0 = f a + f a ′=3.5+3.4 MHz=6.9 MHz, where f S− =( f 0 + f a )− f a ′ and f S+ =( f 0 + f a )+ f a ′ are the downshifted and upshifted frequencies of the sample beam because of the focused ultrasonic modulation at f a ′), which caused the hologram to be washed out. We further validated TRUE focusing by imaging an absorptive target, which was sandwiched between the two scattering media and scanned along the x direction with a step size of 0.2 mm. At each scanning position, to make sure that we indeed obtained signals from TRUE light instead of from R* light that was randomly scattered by the PRC because of beam fanning, a signal was obtained by taking the difference between the peak photodiode outputs corresponding to the two hologram-recording states (that is, focused ultrasound on and off) [19] , [21] , [22] . At each scanning position, 20 TRUE focusing procedures (ultrasonic modulation on and off alternately 10 times during hologram recording) were performed to obtain a 10-time-averaged signal, and the TRUE focusing procedures were operated at a repetition rate of 20 Hz. In each cycle (50.0 ms long), 10.0 ms was used in hologram recording, 0.6 ms was used for completely shutting off the writing beams, 2.0 ms was used in hologram reading and the remaining 37.4 ms was idle (that is, ultrasound was turned off, and shutters were closed) to protect the ultrasonic transducer from overheating by reducing its duty cycle. One-dimensional (1D) images of the target are shown in Fig. 2j , when the IP was static ( τ c >300 s) and when it was moved at a speed of 0.100 mm s −1 ( τ c =5.6 ms). The dips in the images represent the absorptive target, since it absorbed part of the TRUE light. The image qualities for τ c =5.6 ms and τ c >300 s are comparable in terms of target position, dimension, contrast and resolution, demonstrating that focusing was achieved inside a dynamic scattering medium with a speckle correlation time as short as 5.6 ms. The resolution of the image obtained from curve fitting was 0.90 mm (see Methods), which was in agreement with the theoretical value of 0.87 mm, as determined by the focal width of the ultrasonic transducer (3.5 MHz, numerical aperture (NA)=0.25). As a control, when the frequency of the focused ultrasonic modulation was downshifted by 100 kHz relative to its correct value, the target could not be imaged, as expected. Living tissue experiments The capability of our system to tolerate fast speckle decorrelation ( τ c ≥5.6 ms) paves the way to achieve TRUE optical focusing even when the scattering medium is living tissue whose speckle correlation time is in the order of 1 ms, depending on the depth of interest. A 350-μm-thick living-mouse ear (which comprises two skin layers that are fed by separate blood and lymphatic circulations, with a cartilage layer sandwiched in the middle) was used in our experiments. The optical thickness of the mouse ear, defined as the negative natural logarithm of the fraction of unscattered light, was measured to be 17.4±0.1 (see Methods); therefore, the power of the ballistic light component is negligible compared with the total light power (ratio <2.8 × 10 −8 ). In addition, no optical focus could be observed by directly focusing light through a living-mouse ear with a microscope objective (see Supplementary Fig. 3 ). We first measured the speckle correlation time of the ear of a living mouse under normal anaesthesia (see Methods). A sequence of speckle patterns was recorded at 30 fps (see Supplementary Movie 1a ), from which the speckle correlation coefficient was computed and is shown as a function of time in Fig. 3a . The movie shows a fast-decorrelating speckle pattern on top of a slowly decorrelating background speckle pattern (see Supplementary Note 2 for a detailed analysis). The background speckle pattern, presumably mainly formed by photons not scattered by blood, translated 0.64 μm back and forth every 800 ms with a duration of 65 ms, because of the breathing of the mouse. The fast-decorrelating speckle pattern, on the other hand, was possibly mainly formed by photons scattered by blood. To validate this hypothesis, we recorded speckle patterns before and after blocking the blood flow in the mouse ear ( Supplementary Movie 1 ) and employed a faster sCMOS camera (with a frame rate of 2,271 fps at 160 × 38 resolution) to measure the speckle correlation time. The speckle correlation coefficients for five different locations on the mouse ear were computed from movies and are shown as a function of time in Fig. 3b . The value of τ c determined thereby ranges from less than 0.44 ms (limited by the camera’s frame rate) to 10 ms, depending on the measurement position. Given that τ c can be estimated by [43] , [44] τ c ≈ λ / v , where λ is the wavelength of light and v is the blood flow speed, the range of τ c is in accordance with the fact that the flow speed in a mouse ear can range from 0.11 mm s −1 in capillaries [45] to 5.0 mm s −1 in arteries [46] . Once the blood flow was blocked by pressing the ear against a stiff acrylic wall with a metal bar (see Supplementary Fig. 4 ), τ c became much larger (>500 ms, see the top, almost flat curve in Fig. 3b and Supplementary Movie 1b ), confirming that the fast speckle decorrelation was due to the light scattered by blood. 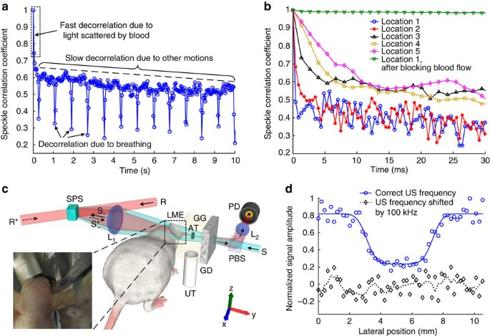Figure 3: TRUE optical focusing inside a dynamic scattering medium containing a living-mouse ear. (a) The speckle correlation coefficient as a function of time for a living-mouse ear. Three speckle decorrelation characteristics were identified. (b) The speckle correlation curves measured at five locations on the mouse ear. The speckle correlation time (τc) determined from the curves ranged from less than 0.44–10 ms. When the blood flow was blocked,τcbecame much larger. (c) Schematic of the set-up for imaging an absorptive target placed between a living-mouse ear and a diffuser. The target was scanned along thexdirection. Inset: a photo showing the right ear of a mouse used as a dynamic scattering medium. The left ear was bent downwards to avoid blocking the light. Aluminium foil tapes were used to block the light that did not pass through the right ear. (d) 1D images of the absorptive target. The circles and diamonds denote experimental data. The solid line denotes curve fitting of the experimental data. The dotted line denotes the four-point moving average of the experimental data. AT, absorptive target; GD, ground glass diffuser; GG, gelatin gel; L, lens; LME, living-mouse ear; PBS, polarizing beamsplitter; PD, photodiode; R, reference beam; R*, reading beam, phase conjugate to R; S, sample light; S−, frequency-downshifted sample light (signal light);, time-reversed signal light; SPS, Sn2P2S6:Te 1% photorefractive crystal; TRUE, time-reversed ultrasonically encoded; US, ultrasound; UT, ultrasonic transducer. Figure 3: TRUE optical focusing inside a dynamic scattering medium containing a living-mouse ear. ( a ) The speckle correlation coefficient as a function of time for a living-mouse ear. Three speckle decorrelation characteristics were identified. ( b ) The speckle correlation curves measured at five locations on the mouse ear. The speckle correlation time ( τ c ) determined from the curves ranged from less than 0.44–10 ms. When the blood flow was blocked, τ c became much larger. ( c ) Schematic of the set-up for imaging an absorptive target placed between a living-mouse ear and a diffuser. The target was scanned along the x direction. Inset: a photo showing the right ear of a mouse used as a dynamic scattering medium. The left ear was bent downwards to avoid blocking the light. Aluminium foil tapes were used to block the light that did not pass through the right ear. ( d ) 1D images of the absorptive target. The circles and diamonds denote experimental data. The solid line denotes curve fitting of the experimental data. The dotted line denotes the four-point moving average of the experimental data. AT, absorptive target; GD, ground glass diffuser; GG, gelatin gel; L, lens; LME, living-mouse ear; PBS, polarizing beamsplitter; PD, photodiode; R, reference beam; R*, reading beam, phase conjugate to R; S, sample light; S − , frequency-downshifted sample light (signal light); , time-reversed signal light; SPS, Sn 2 P 2 S 6 :Te 1% photorefractive crystal; TRUE, time-reversed ultrasonically encoded; US, ultrasound; UT, ultrasonic transducer. Full size image TRUE optical focusing was further demonstrated by imaging an absorptive target embedded between the living-mouse ear and a ground glass diffuser ( Fig. 3c ). By scanning the target along the x direction and monitoring the transmitted TRUE light power at each scanning position, a 1D image of the target was obtained, as shown in Fig. 3d . The target is clearly revealed as a dip with an image resolution of 1.1 mm determined from the curve fitting, which is reasonably close to the size of the ultrasonic focus. As a control, when the frequency of the focused ultrasonic modulation was downshifted by 100 kHz relative to its correct value, the target could not be imaged, as expected. In these experiments, we applied the same averaging scheme as in the phantom experiments. To push the imaging speed, TRUE focusing procedures were operated at 132 Hz at each scanning position, and the transducer ran at a much higher duty cycle than it ran in the experiments with phantoms. The shutters were operated in burst mode. In each TRUE focusing procedure (7.6 ms), 5.0 ms was used in hologram recording, 0.6 ms was used for completely shutting off the writing beams and 2.0 ms was used in hologram reading. The intensity of the reference beam was 1.0 W cm −2 in the dynamic phantom experiment and 1.8 W cm −2 in the living tissue experiment. In both cases, the intensity of the sample light on the crystal was about seven times weaker. We tested different power-splitting ratios between the sample beam and the reference beam, and determined the optimum intensity ratio (1:8) by maximizing the time-reversed signal strength. So far, we have not found a satisfactory theoretical explanation of the optimum intensity ratio. Optical focusing at depths beyond one transport mean free path inside living biological tissue is one of the most challenging goals in biomedical optics. The focusing speeds of the previous internal-guide-star-based wavefront shaping and TRUE focusing techniques are far too low for in vivo applications where the fast speckle decorrelation caused by living tissue needs to be overcome. In this study, we improved the speed of focusing light deep inside scattering media by two orders of magnitude, and provided the first demonstration of using TRUE light to focus inside a dynamic scattering medium comprising living tissue. Since our system uses a near-infrared wavelength, it has the potential to focus light deep inside tissue due to the weaker optical attenuation. The speckle size on the PRC in the dynamic phantom experiment was measured to be 1.6 μm; therefore, the number of optical modes accommodated by the PRC was estimated to be ( A / d ) 2 =(6 × 10 3 /1.6) 2 =1.4 × 10 7 (where A =6 mm is the area of the front surface of the PRC and d =1.6 μm is the speckle size on the PRC), which is 22 times more than that can be accommodated by a state-of-the-art SLM (1,920 × 1,280 pixels) used in digital TRUE focusing systems or wavefront-shaping techniques. The large number of optical modes, N , controlled by our system, enables a more complete phase conjugation [24] and a focus with a higher peak to background ratio [21] , [24] , [25] , [27] (PBR=( N+ 1)/ M , where M is the number of optical modes inside the focus) under the same experimental condition. It will take ~1.9 × 10 3 s to handle the same number of optical modes even using the fastest implementations demonstrated in wavefront shaping [28] , [29] (although the number of pixels in a digital micromirror device [28] or a microelectromechanical deformable mirror [29] is far less than 1.4 × 10 7 ), which is 1.5 × 10 5 times less than the focusing speed of our system. A large N is desired to achieve a sufficient PBR in deep tissue because M can be as large as ~[ λ a /( λ /2/ n )] 2 =[150 μm/(0.8 μm/2/1.33)] 2 =2.5 × 10 5 in the acoustic-wave-guided wavefront shaping (assuming a 10-MHz ultrasonic wave whose wavelength λ a is 150 μm, an optical wavelength λ of 0.8 μm in vacuum, a refractive index n of 1.33 for water in biological tissue and fully developed speckles). We note a recent report [47] on focusing light through a thin dynamic scattering medium having a speckle correlation time as short as 620 ns, by using the self-organization of the optical field inside a multimode laser cavity to generate the optimal wavefront. Despite its superior speed, this technique relies on a pinhole at the targeted location to provide the feedback, preventing it from focusing light noninvasively inside living biological tissue. Moreover, the demonstrated number of controlled optical modes was only ~1,000, and it becomes even smaller for thicker samples as limited by the isoplanatic angle [47] . In the dynamic phantom experiment, we determined the optimum hologram writing time (10 ms) by maximizing the signal-to-noise ratio when τ c =5.6 ms. The shorter speckle correlation time seems to contradict the fact that time-reversal could still be achieved, which, however, can be explained as follows. Although the recorded hologram was partially blurred, it could be decomposed into a correct hologram and an incorrect one. The correct hologram generated a TRUE focus, while the incorrect one produced a background. For the background, light energy was broadly distributed in space so that the intensity was much lower than that in the TRUE focus. Since the hologram-writing time was only 79% longer than τ c and 43% longer than the response time of the PRC [38] , [39] (7 ms at 1 W cm −2 ), the correct hologram still prevailed, forming a TRUE focus (see the simulation results in Supplementary Fig. 5 and Supplementary Note 3 ). In the experiment with living tissue, the light intensity on the mouse ear was 0.42 W cm −2 , which is close to the American National Standards Institute (ANSI) safety limit at ~793 nm (0.30 W cm −2 ). No apparent damage was observed in the tissue after the experiment. It is also worth noting that the ANSI safety limit is usually 10 times below the real damage threshold. Nevertheless, we could further decrease the light intensity on the tissue to meet the standard. By recording the speckle patterns of the light passing through the living-mouse ear, we found that some part of the pattern (mainly formed by blood-scattered light) decorrelated fast ( τ c ranged from less than 0.44 to 10 ms), while the rest (mainly formed by nonblood-scattered light) decorrelated slowly ( τ c >60 s, when the motion of the ear due to breathing was suppressed by a home-made immobilization set-up, which gently pressed the ear using two microscope slides). Since the response time of the PRC is inversely proportional to the illuminating light intensity and the intensity was higher on the PRC in the living tissue experiment than that in the dynamic phantom experiment, we expect our system to have achieved TRUE focusing when τ c was less than 5.6 ms in the living tissue experiment. Considering the range of τ c of a living-mouse ear, we reasoned that most of the nonblood-scattered photons and part of the blood-scattered photons impinging on the PRC were time-reversed back to the acoustic focus. Cui et al . [48] reported light transmission through (as opposed to focusing inside) a living rabbit ear by OPC and measured the speckle correlation time to be 1.5 s. Considering the speed of their system, we believe they time-reversed only the photons that were not scattered by blood, which formed a quasi-static speckle pattern on the camera. For thicker tissue, however, the number of photons that are not scattered by blood becomes smaller, and the photons that are multiply-scattered by blood tend to result in a faster decorrelating speckle pattern [49] . In order to achieve TRUE focusing in these situations, higher speed is needed. To this end, one may boost the reference beam intensity to further decrease the PRC’s response time, which, however, may decrease the TRUE signal amplitude due to a non-optimum intensity ratio between the reference beam and the signal beam on the PRC, once the intensity of the sample beam is limited by the ANSI safety limit. Alternatively, one may employ faster PRCs, such as GaAs [50] . In the future, to achieve TRUE focusing inside thick tissue, we plan to implement the system in a reflection configuration [19] , where light is illuminated and detected on the same side of the tissue. For applications such as photodynamic therapy or multiphoton imaging, where large energy or power deposition is needed, it is important to add gain to the TRUE light. Nevertheless, even without gain, it has been shown that there is enough TRUE light to achieve single-photon fluorescence imaging [21] deep inside scattering media. To conclude, we focused diffuse light inside a dynamic scattering medium containing either a tissue-mimicking phantom or living tissue. Our system can tolerate rapid speckle decorrelation on the scale of 5.6 ms. Because the demonstrated focusing speed approaches the tissue decorrelation rate, this work is an important step towards in vivo deep tissue optical imaging, manipulation, optogenetics and photodynamic therapy. Sample preparation The intralipid–gelatin phantom was made from intralipid (Intralipid 20%, Fresenius Kabi, Sweden), porcine skin gelatin (10% by weight, no. G2500-1kG, gel strength 300, Sigma-Aldrich, USA) and de-ionized water [51] with a lipid concentration of 1.5 g ml −1 . The reduced scattering coefficient μ S ′ was measured by a home-built oblique incidence reflectometer [52] to be 9.8 cm −1 . Acrylic spacers with a thickness of 1.5 mm were sandwiched between two acrylic sheets to accurately control the thickness of the intralipid–gelatin phantom to be 1.5 mm (equivalent to 1.5 l t ′). The clear gelatin-gel layer was made from porcine skin gelatin (10% by weight) and de-ionized water. The optical absorptive target (3.9 mm × 1.3 mm × 20.0 mm along the x , y and z directions) was made from black ink, gelatin and distilled water. The absorption coefficient of the target was 0.80 cm −1 , as measured by a spectrophotometer (Cary Eclipse, Varian, USA). The diffuser (DG20-120, Thorlabs, USA) was embedded inside the gelatin gel to position it closer to the absorptive target (distance=8.0 mm) and the intralipid–gelatin layer (distance=22.1 mm) without blocking the ultrasonic waves. Experimental set-up The experimental set-up for imaging the absorptive target with TRUE light is schematically shown in Supplementary Fig. 1 . The light source was a 1.6-W continuous-wave Ti:Sapphire laser (MBR 110, Coherent, USA) operating at 793 nm, pumped by a 532-nm continuous-wave laser (Verdi 10, Coherent). A TRUE focusing procedure consisted of recording and reading a hologram. In the recording phase, the laser output was switched to horizontal polarization by an electro-optic modulator (EOM, 350-80-LA-02, Conoptics, USA) to transmit through the first polarizing beamsplitter (PBS1). The residual light reflected from PBS1 was completely blocked by a mechanical shutter MS2 (Uniblitz LS3, Vincent Associates, USA). The transmitted light was split into a sample beam and a reference beam by PBS2, with a splitting ratio controlled by the second half-wave plate. The sample beam S passed through two AOMs (IntraAction AOM-802AF1) to achieve a frequency shift to f = f 0 + f a , where f 0 was the laser frequency and f a (3.5 MHz) was the frequency shift due to the two AOMs (shifted by +75 and −71.5 MHz, respectively). A function generator (33250A, Agilent, USA) sent a 150-mVpp sinusoidal wave with a frequency of f a to a 50-dB gain RF power amplifier (325LA, ENI, USA) to drive the spherically focused ultrasonic transducer (A381S 3.5 MHz, Panametrics, USA). Owing to the acousto-optic effect, a small portion of the light traversing the acoustic focus was frequency-shifted to f 0 and f 0 +2 f a . Only the frequency-downshifted (that is, at f 0 ) sample light (also called signal light) S − and the reference beam R contributed to a stable hologram in the Sn 2 P 2 S 6 :Te 1% crystal (6 × 6 × 6 mm 3 ). When interfering with R, the sample light at frequency f 0 + f a (or f 0 +2 f a ) formed a beat with a frequency of f a (or 2 f a ), which was too fast for the crystal to respond to and the hologram was washed out. The R and S beams illuminated the PRC at about ±11 degrees from the normal of the PRC surface for 10 and 5 ms in the dynamic phantom and the living tissue experiments, respectively. In the hologram reading phase, the laser light was switched to vertical polarization by the EOM and reflected by PBS1 to form the reading beam R*, which was phase-conjugated to R. The residual horizontally polarized light transmitted through PBS1 was blocked by the shutter MS1. When the 3.4-W cm −2 R* beam illuminated the PRC, the time-reversed signal light was generated and converged back to the acoustic focus. A portion of was then reflected by PBS3 and detected by a photodiode (PDA36A, Thorlabs, USA) with a 70-dB gain. The signal was digitized by an oscilloscope (TDS 5034, Tektronix, USA) running in fast frame mode and sent to a PC via a GPIB cable and a GPIB-USB controller. The ultrasound was off during the hologram-reading phase. Although R* was on for 2 ms (the minimum exposure time determined by the mechanical shutter), the maximum signal amplitude was detected by the photodiode immediately after the shutter MS2 was opened since the signal decayed quickly as the hologram was being washed out by the reading beam. The intralipid–gelatin phantom was mounted on a linear stage (462-X-M, Newport, USA) driven by a motorized actuator (CONEX-TRA25CC, Newport) to control the movement speed. The timing of the EOM, shutters and function generators was controlled by a pulse delay generator (DG645, Stanford Research Systems, USA), which was externally triggered by a multifunction DAQ (NI USB-6008, National Instruments, USA) controlled by a PC. Measurement of the speckle correlation time of the sample To measure the speckle correlation time ( τ c ) of the dynamic phantom, we used a CMOS camera (208 fps, 320 × 108 pixels, global shutter, exposure time=0.062 ms, FMVU-03MTM, Point Grey, Canada) to record the speckle patterns magnified by an objective (× 40, NA=0.65, tube length=160 mm, Leica E 1 ACHRO; Fig. 2a ). The NA of the objective was chosen to be greater than the image space NA of lens L (0.23) in Fig. 2a,d,i (composed of L3 and L4, see Supplementary Fig. 1 ), so that it did not restrict the NA of the system. Otherwise, τ c cannot be measured correctly since it is inversely proportional to the NA of the objective when NA<0.23, which was proved in theory and verified by our experiments using objectives with different NA (data not shown). To measure τ c of the living tissue, we illuminated the left mouse ear (sandwiched between a cover slip (thickness=0.17 mm, VWR 48393-172) and a microscope slide (thickness=1 mm, Corning 2947-75 × 25)) with a beam 5.0 mm in diameter; the large vessels in the centre were covered by the beam. The other mouse ear was bent downwards and taped to the home-built animal holder to avoid blocking the light. During the experiment, the mouse (15-week-old, Female, Hsd:Athymic Nude-Foxl NU, Harlan Co., USA) was held on a heating pad (SRFG-104/10, Omega, USA) whose temperature was set to 37 °C by a controller (YO-89802-52, Cole-Parmer, USA) to maintain the mouse’s body temperature. This temperature was crucial to keep a normal blood flow speed. The mouse was held steady with a home-machined hard palate fixture and kept still by using a breathing anaesthesia system (E-Z Anesthesia, Euthanex, USA). All experimental animal procedures were carried out in conformity with the laboratory animal protocol approved by the Animal Studies Committee at Washington University in St Louis. At first, a CMOS camera (30 fps, 344 × 216 pixels, global shutter, exposure time=0.062 ms, FMVU-03MTM, Point Grey) was used to record the speckle patterns magnified by an objective (× 60, NA=0.80, tube length=160 mm, Nikon, Japan). Then, a faster sCMOS camera (pco. Edge, PCO AG, Germany) was used to record speckle patterns at a higher frame rate (2,271 fps, 160 × 38 pixels, global shutter, exposure time=0.010 ms), from which we obtained τ c of a living-mouse ear. We shifted the positions of the objective and the camera to record the speckle patterns at five different locations on the mouse ear. To block the blood flow, a metal bar pressed the ear against a stiff acrylic wall. We monitored the speckle patterns from 20 s till 12 min after blocking the blood flow, and no fast-decorrelating (on a time scale of 1–10 ms) speckle patterns were observed. Determination of the image resolution Since the 1D point spread function of the system can be approximated by a Gaussian function PSF( x )= A exp (− x 2 /2 σ 2 ), and the transmission of the object (whose boundary positions are specified by x 1 and x 2 ) can be approximated by a rectangular function o( x )=− B [u ( x − x 1 )−u ( x−x 2 )], the 1D image of the object can be written theoretically as a convolution: , where A , B and C are constants, u ( x ) is the step function and is the error function. By fitting the experimental data with , we obtained σ , which was related to the image resolution (defined as the full-width at half maximum of the Gaussian profile) as in . Measurement of the optical thickness of a living-mouse ear We illuminated the living-mouse ear perpendicularly with a collimated laser beam (beam width ~1.5 mm) and measured the power of the transmitted ballistic light at 2 m away [25] , [53] from the ear using a photodiode (PDA36A, Thorlabs, USA) to be (2.8±0.3) × 10 −8 of the power of the incident light. Thus, the optical thickness of the mouse ear, defined as the negative natural logarithm of the fraction of unscattered light, was measured to be 17.4±0.1 (for six mice). All mice were under anaesthesia during the measurement. Simulation methods Here we describe the simulation methods to obtain the results shown in Fig. 1b–e . Inside the scattering media, the two-dimensional (2D) light field on the x–z plane intersecting the acoustic axis (denoted as plane A, see Fig. 1a ) was represented by a random complex matrix A 0 (dimension=40 × 40), whose elements followed the circular Gaussian distribution [24] , [54] . Upon ultrasonic modulation, the light field became A=A 0 × I US , where ‘ × ’ represents element-wise multiplication, and I US is the 2D acoustic intensity distribution on plane A, approximated by (see Supplementary Fig. 5k ). is a constant, , , where NA is the numerical aperture of the transducer, and λ is the acoustic wavelength. A was then reshaped to a column vector a with a dimension of 1,600 × 1. Propagation of the ultrasonically encoded light through the scattering medium and the free space was simulated by multiplying a with a transmission matrix [14] , [55] T (dimension=1,600 × 1,600). In our experiment, the number of modes on the PRC was much smaller than the total number of output modes. Under this condition, the elements of T obeyed the circular Gaussian distribution [24] . The signal light field on the PRC was calculated by b = Ta . To simulate dynamic scattering media, we generated 51 independent random matrices T i ( i =0, 1, 2, , 50, representing the scattering medium at the time of i ms), whose elements followed the circular Gaussian distribution and , where ‘†’ denotes conjugate transpose and is the identity matrix. Since different matrices T i were uncorrelated, b i = T i a were uncorrelated; therefore, the speckle correlation time τ c was smaller than 1 ms. The signal light b i interfered with a reference beam R (whose electric field was represented by a vector R (dimension=1,600 × 1) in which all elements were 1), and formed an interference pattern I i =| b i + R | 2 on the PRC. The hologram recorded on the PCM at time t can be calculated by [56] , where τ r is the response time of the PCM. We let and denote the response times of a fast PCM and a slow PCM, and assumed and . Therefore, at t =50 ms, the hologram recorded in a slow PCM (shown in Fig. 1b ), h s , was approximately proportional to (and simulated by) (since ), and the hologram recorded in a fast PCM (shown in Fig. 1c ), h f , was approximately proportional to (and simulated by) I 50 =| b 50 + R | 2 (since ). In the time-reversal step, the holograms h s and h f were read by R* (whose electric field was represented by a vector R *) at t =50 ms, and the −1st order diffracted light was proportional to and , respectively. At this time, the dynamic scattering medium was represented by the transmission matrix T 50 ; therefore, on plane A, the light field distribution for the slow PCM and (since ) for the fast PCM, where the superscript ‘ ’ denotes matrix transpose. It can be seen that resembles the perfect time-reversed light field a * The intensity distributions shown in Fig. 1d,e were calculated by and with bicubic interpolation. How to cite this article: Liu, Y. et al . Optical focusing deep inside dynamic scattering media with near-infrared time-reversed ultrasonically encoded (TRUE) light. Nat. Commun. 6:5904 doi: 10.1038/ncomms6904 (2015).